PFKFB4 controls embryonic patterning via Akt signalling independently of glycolysis How metabolism regulators play roles during early development remains elusive. Here we show that PFKFB4 (6-phosphofructo-2-kinase/fructose-2,6-bisphosphatase 4), a glycolysis regulator, is critical for controlling dorsal ectoderm global patterning in gastrulating frog embryos via a non-glycolytic function. PFKFB4 is required for dorsal ectoderm progenitors to proceed towards more specified fates including neural and non-neural ectoderm, neural crest or placodes. This function is mediated by Akt signalling, a major pathway that integrates cell homeostasis and survival parameters. Restoring Akt signalling rescues the loss of PFKFB4 in vivo . In contrast, glycolysis is not essential for frog development at this stage. Our study reveals the existence of a PFKFB4–Akt checkpoint that links cell homeostasis to the ability of progenitor cells to undergo differentiation, and uncovers glycolysis-independent functions of PFKFB4. Embryonic patterning involves the complex interplay of multiple signalling pathways triggering gene regulatory networks, which, in turn, drive cell-fate choices and progenitor cell differentiation. While cancer cell metabolism is linked to cancer progression [1] , [2] , [3] , [4] , [5] , [6] , it remains unknown whether the homeostatic balance of progenitor cells affects their ability to undergo differentiation programmes. In particular, the cell metabolic status, its proliferative state and the activity of survival pathways could be important checkpoints for cell patterning progression during development. PFKFB1–4, a highly conserved family of bifunctional kinases/phosphatases, optimizes the cellular rate of glycolysis [7] , [8] . We found that pfkfb4 expression is enriched at the dorsal side of frog and chick embryos during early development [9] . However, glucose is not the main source of energy in embryos: the early frog embryo uses yolk-derived amino acids to fuel directly the citric acid cycle in the mitochondria [10] , [11] . This raised the intriguing possibility that PFKFB4 could play novel roles in dorsal ectoderm formation, besides its classical function on glycolysis regulation. Here, we demonstrate that PFKFB4 levels control the switch of immature ectoderm progenitors towards specified dorsal fates, including neural plate, neural crest, placodes and non-neural ectoderm, in a glycolysis-independent manner. In contrast, we find that PFKFB4 regulates Akt phosphorylation in vivo , that the drug-mediated inhibition of Akt phenocopies the PFKFB4 morphant phenotype and that Akt activation rescues the patterning defects in morphant embryos. As PFKFB4-dependent Akt signalling is essential for the progression of embryonic patterning, we propose that PFKFB4 is a pivotal and multifunctional regulator linking cell homeostasis and survival to progenitor cell patterning. PFKFB4 is essential for dorsal ectoderm development During vertebrate gastrulation and neurulation, the dorsal ectoderm is patterned into several cell fates: neural plate (NP), non-neural ectoderm (NNE), neural crest (NC) and preplacodal ectoderm (P), a prerequisite for the differentiation of the central and peripheral nervous systems and surrounding tissues. Focusing on genes enriched dorsally during neurulation [9] , [12] , we found that expression of pfkfb4 (6-phosphofructo-2-kinase/fructose-2,6-bisphosphatase isoform-4), gene coding a key regulator of glycolysis [7] , [8] ( Supplementary Fig. 1 ), was increased in dorsal ectoderm during gastrulation and neurulation in frog and chick embryos ( Fig. 1a,b ; Supplementary Fig. 2 ). Pfkfb4 late gastrula expression overlapped with the pattern of the neurectoderm marker sox2 ; while pfkfb4 mid-neurula expression was restricted to the anterior neural folds, similar to neural border ( zic1, pax3) and NC ( snail2 ) markers, with a faint NP expression ( Fig. 1a,b ; Supplementary Fig. 2 ) [13] . Pfkfb4 is the major isoform in dorsal tissues [9] . To address the role of PFKFB4, we validated pfkfb4 translation and splice-blocking morpholinos (ATG/SP-MO, Fig. 1c,d ; Supplementary Fig. 3 ). Morphant embryo morphology was normal until mid-neurula (stage 14), then the injected cells underwent a marked cell apoptosis and embryos died at late neurula stage (stage 18–20, Fig. 1e ). This striking phenotype was strictly dependent on PFKFB4 depletion as a ‘rescue’ experiment, using coinjection of pfkfb4 SP-MO with pfkfb4 -encoding mRNA (messenger RNA) (insensitive to the morpholino), abolished cell death and restored normal development ( Fig. 1e ; 90% of morphants show increased cell death at stage 14, whereas only 45% of embryos do in the rescue situation). We concluded that PFKFB4 activity was essential for dorsal ectoderm survival during neurulation. 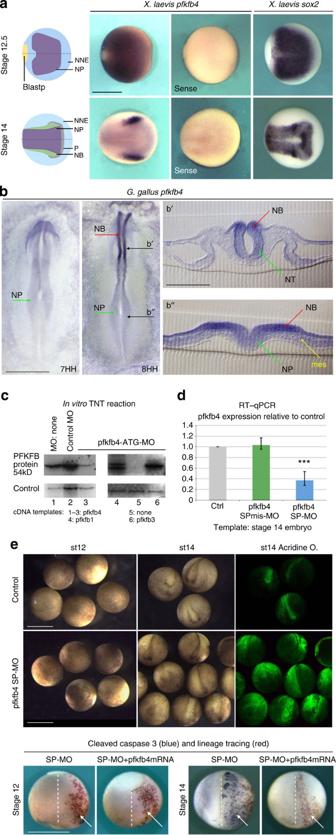Figure 1:Pfkfb4is enriched in the developing dorsal ectoderm and is required for its survival during neurulation. (a) Dorsal ectoderm territories are schematized inX. laevislate gastrulas (stage 12.5) and mid-neurulas (stage 14): non-neural ectoderm (NNE), neural plate (NP), neural border (NB), preplacodal ectoderm (P) and blastopore (Blastp). In late gastrulas,pfkfb4is expressed broadly dorsally, encompassingsox2pan-neural expression. Later,pfkfb4is weak in the NP and enriched at the NB,sox2marks the NP. WISHs are shown with antisense and control sense probes. Scale bar, 1 mm. Additional views are shown inSupplementary Fig. 2. (b)pfkfb4is similarly enriched in the NP ofG. galluslate gastrulas (stage 6–7HH) and NB of early neurulas (stage 8HH). In contrast, mesoderm (mes) is barely stained as seen on stage 8HH chick transverse sections (b′,b″). Scale bars, (b: 1 mm) (b′,b″: 0.3 mm). (c) Translation-blockingpfkfb4ATG-MO specifically decreases PFKFB4 protein synthesis usingin vitrotranscription and translation (TNT) assay, from cDNA template. (d) Splice-blockingpfkfb4MO depletes endogenouspfkfb4mRNAin vivo(RT–qPCR).Pvalues were generated using ANOVA test (P<0.001) and error bars represent s.e.m. Controls include control MO (candd),pfkfb1orpfkfb3cDNA templates (c). At least three independent experiments were performed. (e) PFKFB4 morphant phenotype: morphology and cell death analysis by acridine orange staining (green staining) and activated caspase-3 immunostaining (blue staining), (14 independent experiments, a total of 649 embryos were analysed and detailed statistical analysis is available inSupplementary Table 2). While morphant embryos undergo marked cell death in the injected area after stage 13–14, restoringpfkfb4 mRNA rescues the death phenotype (8% of embryos show dead cells before stage 13; 90% of morphant embryos with increased cell death at stage 14 (10% normal embryos); only 45% of embryos with dead cells at stage 14 afterpfkfb4mRNA coinjection (55% normal embryos as depicted). Arrows mark the injected cells, traced using beta-galactosidase staining (in red, see Methods). Figure 1: Pfkfb4 is enriched in the developing dorsal ectoderm and is required for its survival during neurulation. ( a ) Dorsal ectoderm territories are schematized in X. laevis late gastrulas (stage 12.5) and mid-neurulas (stage 14): non-neural ectoderm (NNE), neural plate (NP), neural border (NB), preplacodal ectoderm (P) and blastopore (Blastp). In late gastrulas, pfkfb4 is expressed broadly dorsally, encompassing sox2 pan-neural expression. Later, pfkfb4 is weak in the NP and enriched at the NB, sox2 marks the NP. WISHs are shown with antisense and control sense probes. Scale bar, 1 mm. Additional views are shown in Supplementary Fig. 2 . ( b ) pfkfb4 is similarly enriched in the NP of G. gallus late gastrulas (stage 6–7HH) and NB of early neurulas (stage 8HH). In contrast, mesoderm (mes) is barely stained as seen on stage 8HH chick transverse sections ( b ′, b ″). Scale bars, ( b : 1 mm) ( b ′, b ″: 0.3 mm). ( c ) Translation-blocking pfkfb4 ATG-MO specifically decreases PFKFB4 protein synthesis using in vitro transcription and translation (TNT) assay, from cDNA template. ( d ) Splice-blocking pfkfb4 MO depletes endogenous pfkfb4 mRNA in vivo (RT–qPCR). P values were generated using ANOVA test ( P <0.001) and error bars represent s.e.m. Controls include control MO ( c and d ), pfkfb1 or pfkfb3 cDNA templates ( c ). At least three independent experiments were performed. 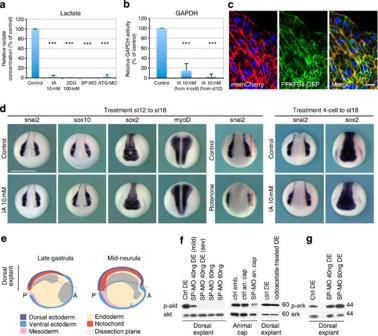Figure 2: PFKFB4 controls Akt signallingin vivo, independently of glycolysis regulation. (a,b) Lactate concentration (a) and GAPDH activity (b) confirmed glycolysis blockade with 2DG (100 mM) or IA (10 mM) (% of control sample value, 9 independent experiments with 10 embryos for each condition in each experiment; Student’st-test:P<0.001. Error bars represent s.d.). Similar dosage in PFKFB4 morphants also shows efficient glycolysis blockade. (c) Subcellular localization of PFKFB4–GFP in dorsal ectoderm cells was restricted to the cytoplasm (membranetagged-cherry-fp, pfkfb4–gfpinjections, with nuclear DAPI staining, transverse section through neural plate, neural crest and ectoderm). Scale bar, 15 μm. (d) Normal neurula patterning occurred when glycolysis was blocked by IAin vivo, either from four-cell stage to stage 18, or during neurulation (st12-st18) (similar results were obtained with 2DG, as shown inSupplementary Fig. 4). In contrast, a short treatment with the mitochondrial blocker rotenone (0.05 μM) rapidly stopped neurulation and patterning. Scale bar, 1 mm. (e) Dorsal explants (DE) were dissected from either late gastrula (stage 12) or mid-neurula (stage 14) embryos (schematic sagittal view with dissection plane as dotted line, A; anterior, P; posterior). (f) Akt phosphorylation was decreased in DE or in animal caps (AC) followingpfkfb4SP-MO injection at increasing doses (40 ng—embryos were sorted according to their mild or severe phenotype— or 60 ng). Akt phosphorylation was unchanged after glycolysis blockade. (g) Erk phosphorylation was present in DE followingpfkfb4SP-MO injection. (f,g) At least three independent experiments were performed for each condition, all embryos from the same condition presented similar phenotypes as pictured. ( e ) PFKFB4 morphant phenotype: morphology and cell death analysis by acridine orange staining (green staining) and activated caspase-3 immunostaining (blue staining), (14 independent experiments, a total of 649 embryos were analysed and detailed statistical analysis is available in Supplementary Table 2 ). While morphant embryos undergo marked cell death in the injected area after stage 13–14, restoring pfkfb 4 mRNA rescues the death phenotype (8% of embryos show dead cells before stage 13; 90% of morphant embryos with increased cell death at stage 14 (10% normal embryos); only 45% of embryos with dead cells at stage 14 after pfkfb4 mRNA coinjection (55% normal embryos as depicted). Arrows mark the injected cells, traced using beta-galactosidase staining (in red, see Methods). Full size image Glycolysis blockade does not phenocopy PFKFB4 depletion In frog embryos, energy metabolism is mainly driven by amino acids fuelling the Krebs cycle until gastrulation [10] , [11] . However, vertebrate PFKFB enzymes are bifunctional kinases/phosphatases controlling fructose-6-phosphate reversible transformation into fructose-2,6-bisphosphate, a potent allosteric activator of the glycolysis rate-limiting enzyme phosphofructokinase-1 (PFK1, Supplementary Fig. 1 ) [14] , [15] , [16] , [17] . By controlling fructose-2,6-bisphosphate levels, PFKFBs regulate PFK1 activity, thereby controlling glycolysis rate [7] , [8] . Our observation of a key function for PFKFB4 in embryonic cell survival raised two non-exclusive hypotheses: either glycolysis played a specific function in dorsal ectoderm during neurulation or PFKFB4 played a non-metabolic role during dorsal development. To test the first hypothesis, we blocked glycolysis by two distinct pharmacological agents: 2-deoxyglucose (2DG, blocks glycolysis upstream of PFK1) or iodoacetate (IA, inhibits GAPDH activity downstream of PFK1 (ref. 18 )) ( Supplementary Fig. 1 ). Glycolysis was efficiently blocked in vivo , by 2DG, IA or pfkfb4 morpholinos ( Fig. 2a,b ; Supplementary Table 2 ). However, when embryos were treated with 2DG or IA, either from four-cell stage to late neurula stage (that is, reproducing the timing of morpholino injections) or only during neurulation, the embryos developed normally: their external morphology, the expression of NP, NC and paraxial mesoderm markers were normal ( Fig. 2d ; Supplementary Figs 4 and 8 ). No cell death was observed. In contrast, when the mitochondrial blocker rotenone was applied, rapid development arrest was observed: neural tube closure failed and gene expression was blocked (for example, snail2 in NC, Fig. 2d ). The embryos died rapidly. This indicated that embryo energy metabolism is mainly oxidative until neurulation, as reported for earlier cleavage stages [10] . Therefore, as dorsal ectoderm development proceeded normally when glycolysis was blocked, we concluded that the cell death observed after PFKFB4 depletion was not caused by insufficient glycolysis rate. Figure 2: PFKFB4 controls Akt signalling in vivo , independently of glycolysis regulation. ( a , b ) Lactate concentration ( a ) and GAPDH activity ( b ) confirmed glycolysis blockade with 2DG (100 mM) or IA (10 mM) (% of control sample value, 9 independent experiments with 10 embryos for each condition in each experiment; Student’s t -test: P <0.001. Error bars represent s.d.). Similar dosage in PFKFB4 morphants also shows efficient glycolysis blockade. ( c ) Subcellular localization of PFKFB4–GFP in dorsal ectoderm cells was restricted to the cytoplasm (membrane tagged-cherry-fp, pfkfb4–gfp injections, with nuclear DAPI staining, transverse section through neural plate, neural crest and ectoderm). Scale bar, 15 μm. ( d ) Normal neurula patterning occurred when glycolysis was blocked by IA in vivo , either from four-cell stage to stage 18, or during neurulation (st12-st18) (similar results were obtained with 2DG, as shown in Supplementary Fig. 4 ). In contrast, a short treatment with the mitochondrial blocker rotenone (0.05 μM) rapidly stopped neurulation and patterning. Scale bar, 1 mm. ( e ) Dorsal explants (DE) were dissected from either late gastrula (stage 12) or mid-neurula (stage 14) embryos (schematic sagittal view with dissection plane as dotted line, A; anterior, P; posterior). ( f ) Akt phosphorylation was decreased in DE or in animal caps (AC) following pfkfb4 SP-MO injection at increasing doses (40 ng—embryos were sorted according to their mild or severe phenotype— or 60 ng). Akt phosphorylation was unchanged after glycolysis blockade. ( g ) Erk phosphorylation was present in DE following pfkfb4 SP-MO injection. ( f , g ) At least three independent experiments were performed for each condition, all embryos from the same condition presented similar phenotypes as pictured. Full size image PFKFB4 controls Akt phosphorylation in vivo To address the mechanism of PFKFB4-induced cell survival, we hypothesized that PFKFB4 depletion impaired Akt signalling, a critical player in cell survival [19] , [20] . We compared the levels of Akt S473-phosphorylation in control or morphant dorsal explants (DE) ( Fig. 2e,f ). Morphant DE displayed a strong, dose-dependent, reduction of Akt phosphorylation. Similarly, blastula roof ectoderm (animal cap ectoderm) injected with pfkfb4 morpholino displayed reduced Akt phosphorylation. In contrast, Akt phosphorylation was normal in IA-treated DE, indicating that glycolysis inhibition does not affect Akt signalling. To identify other potential perturbations in cell signalling and homeostasis after PFKFB4 depletion, we performed a global kinome analysis, using peptide arrays for 288 serine/threonine and tyrosine kinases [21] : no significant perturbation of main kinase activities was detected. Accordingly, we did not detect major changes in MAPK activation on PFKFB4 depletion in DE ( Fig. 2g ). Finally, as other glycolysis enzymes play roles in the nucleus [22] , [23] , we analysed PFKFB4 subcellular localization. PFKFB4–GFP fusions were injected in mild gain-of-function conditions in vivo . PFKFB4–GFP fluorescence intensity was quantified on NP sections, and compared with control GFP intensity. PFKFB4–GFP was located in the cytoplasm, no nuclear enrichment was seen ( Fig. 2c , Supplementary Fig. 5 ). Altogether, we concluded that a major molecular consequence of PFKFB4 depletion was the defective activation of the Akt pathway, leading to morphant cell death. These data uncover the first glycolysis-independent role for PFKFB enzymes. PFKFB4 controls early neurula dorsal ectoderm specification We then addressed the role of this novel PFKFB4/Akt pathway in developing embryos. We first investigated why PFKFB4 depletion caused such marked embryonic death, by analysing morphant development before cell death. In early neurulas, critical patterning events define the prospective neural tube, NC and placodes from the NNE. Blocking patterning cues in vivo , for example, bone morphogenetic proteins, FGF or Wnt signals, does not result in cell death, but rather in increasing one cell fate at the expense of another [24] , [25] . However, we hypothesized that a global patterning defect, which would not allow alternative fate choice, would eventually result in cell apoptosis. We thus analysed the identity of the PFKFB4 morphant cells, before cell death ( Fig. 3 ). At mid-neurulation (stage 14), unilateral morpholino injections showed increased expression of neural border progenitor markers (compare injected and control sides): zic1 showed robust expansion, pax3 was more modest ( Supplementary Table 2 ). In contrast, markers for specified NP ( sox2) , NC ( snail2 and sox10) , placodes ( six1) and NNE ( epidermal keratin, ep.ker. ), were absent in morphant areas ( Fig. 3a–c , Supplementary Figs 3 and 8 ). This phenotype was efficiently rescued in vivo by restoring PFKFB4 activity in morphants ( Fig. 3d , Supplementary Table 2 ). We confirmed these results using an ex vivo model of neural border and NC induction [26] . Both pax3 and snail2 were efficiently induced by activating Wnt signalling and inhibiting bone morphogenetic protein signalling in blastula ectoderm/animal cap assay [27] . In contrast, in the presence of pfkfb4 morpholino, while pax3 was activated, snail2 induction was defective ( Fig. 3e ). Altogether, these results indicated a global failure to specify both neural and non-neural dorsal ectoderm fates during early neurulation, before apoptosis. In contrast, the expression of markers for neural border progenitors [28] was either unaffected or enlarged. This suggested that earlier modulation of gene expression in immature ectoderm cells may account for the phenotype observed during neurulation. We further analysed the initiation of dorsal progenitors specification during gastrulation, that is, 18 h earlier. While sox2 failed to be induced in the NP, zic1 , a direct target of organizer signals [29] , was normal or expanded ( Fig. 3f , Supplementary Table 2 ). In addition, the maternal gene sox3 was normal until mid-neurula stage ( Fig. 3f ) and the NNE progenitor marker foxi1e was precociously activated (early gastrulation), then ectopically expressed (late gastrulation, Fig. 3f ). Paraxial mesoderm progenitor development ( myod) was roughly normal ( Fig. 3f ). Finally, quantitative PCR with reverse transcription (RT–qPCR) analysis of morphant DE also showed increased progenitor marker expression ( zic1, hes4 and foxi1e ) and decreased specification marker expression ( snail2, sox2 and six1 ), when compared with control ( Fig. 3g ). The global level for the non-neural ectoderm marker ep.ker. was not as significantly decreased at stage 14 ( Supplementary Table 2 ). Collectively, these data demonstrate that PFKFB4 activity is essential for the progression from a progenitor cell status towards specified ectoderm fates in vivo . In addition, when this activity is impaired, it is followed by arrest in the developmental cascade of gene expression (developmental arrest, around stages 10.5–12), then, several hours later, by apoptosis (around stage 14–15). 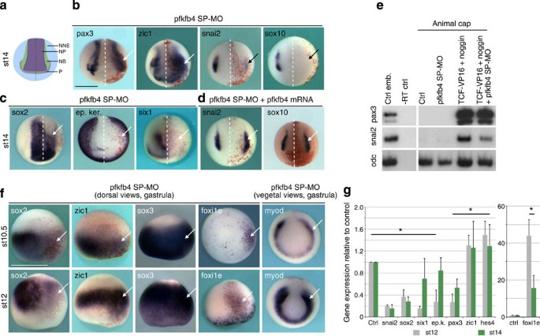Figure 3: Pfkfb4 depletion blocks the early specification of dorsal ectoderm derivatives. (a) Dorsal ectoderm-derived territories at mid-neurulation (stage 14, NNE, NB, NP, P as inFig. 1a). (b,c) PFKFB4 morphant phenotype at mid-neurulation on NB (NC progenitors,pax3andzic1), early NC (snail2andsox10) and on NP (sox2), NNE (ep. ker.) and P (six1). A total of 998 embryos were analysed; the main phenotype is shown and a detailed statistical analysis is given inSupplementary Table 2. Dotted line indicates the mid-line, non-injected side on the left, injected side on the right (arrow, red dots indicate beta-galactosidase lineage tracing). Scale bar, 1 mm. (d)Pfkfb4SP-MO patterning phenotype was efficiently rescued by adding morpholino-insensitivepfkfb4 mRNA. (e) Animal caps were induced to form NB and NC using Wnt activation (with TCF3-VP16) and bone morphogenetic protein blockade (with noggin). Similarly, PFKFB4 knockdown blocked NC induction (snail2), but not NB induction (pax3). (f) Ectoderm patterning defects arise as gastrulation is initiated (stage 10.5) in PFKFB4 morphants:sox2fails to be induced whilemyodremains roughly normal, in contrast, maternal genes and progenitor markers are maintained, expanded or activated ectopically (sox3,zic1, andfoxi1e). (g) RT–qPCR quantification of specification markers (snail2, sox2, six1, andep.ker.)and progenitor markers (pax3,zic1, hes4andfoxi1e) in PFKFB4 morphant embryos, relative to control, during neurulation.Foxi1eshowed very high differential levels in morphant DE compared with controls, asfoxi1eexpression, normally excluded from the dorsal side50, is retained in morphants. Analysis in whole embryos results in increased levels similar to whole-embryo pharmacological treatments (Fig. 4). At least three independent experiments were performed. At-test was used to generate thePvalue (P≤0.01) and error bars represent s.e.m. Figure 3: Pfkfb4 depletion blocks the early specification of dorsal ectoderm derivatives. ( a ) Dorsal ectoderm-derived territories at mid-neurulation (stage 14, NNE, NB, NP, P as in Fig. 1a ). ( b , c ) PFKFB4 morphant phenotype at mid-neurulation on NB (NC progenitors, pax3 and zic1 ), early NC ( snail2 and sox10 ) and on NP ( sox2 ), NNE ( ep. ker .) and P ( six1 ). A total of 998 embryos were analysed; the main phenotype is shown and a detailed statistical analysis is given in Supplementary Table 2 . Dotted line indicates the mid-line, non-injected side on the left, injected side on the right (arrow, red dots indicate beta-galactosidase lineage tracing). Scale bar, 1 mm. ( d ) Pfkfb4 SP-MO patterning phenotype was efficiently rescued by adding morpholino-insensitive pfkfb4 mRNA . ( e ) Animal caps were induced to form NB and NC using Wnt activation (with TCF3-VP16) and bone morphogenetic protein blockade (with noggin). Similarly, PFKFB4 knockdown blocked NC induction ( snail2 ), but not NB induction ( pax3) . ( f ) Ectoderm patterning defects arise as gastrulation is initiated (stage 10.5) in PFKFB4 morphants: sox2 fails to be induced while myod remains roughly normal, in contrast, maternal genes and progenitor markers are maintained, expanded or activated ectopically ( sox3 , zic1 , and foxi1e ). ( g ) RT–qPCR quantification of specification markers ( snail2, sox2, six1 , and ep.ker.) and progenitor markers (pax3, zic1, hes4 and foxi1e ) in PFKFB4 morphant embryos, relative to control, during neurulation. Foxi1e showed very high differential levels in morphant DE compared with controls, as foxi1e expression, normally excluded from the dorsal side [50] , is retained in morphants. Analysis in whole embryos results in increased levels similar to whole-embryo pharmacological treatments ( Fig. 4 ). At least three independent experiments were performed. A t -test was used to generate the P value ( P ≤0.01) and error bars represent s.e.m. Full size image Akt acts downstream of PFKFB4 in dorsal development As PFKFB4 depletion affected Akt phosphorylation, we tested the consequences of Akt signalling inhibition on ectoderm specification in vivo , using the PI3-kinase pharmacological inhibitor LY294002 (ref. 30 ). As early treatments blocked gastrulation as previously reported [30] , we treated embryos with increasing doses shortly after dorsal blastopore lip formation until early or mid-neurula stage ( Fig. 4a,b ). Akt phosphorylation blockade was monitored by western blotting. As in PFKFB4 morphants, both using whole-mount in situ hybridization (WISH) and RT–qPCR, we observed severe loss of snail2 , defective sox2, six1 and ep. ker. expression, and elevated levels of zic1, hes4 and foxi1e ( Fig. 4a,b ; Supplementary Fig. 8 ). Although minor differences were observed in the intensity and timing of gene modulations (see hes4 late increase), the phenotype of PFKFB4 morphants and LY294002-treated neurulas was thus similar. We further compared the effects of PFKFB4 and Akt gain-of-function in vivo : in both cases, very mild NP and NC expansions were observed while NNE was normal ( Fig. 4c ), indicating that neither PFKFB4 nor Akt increased levels modified significantly fate choices in dorsal ectoderm. 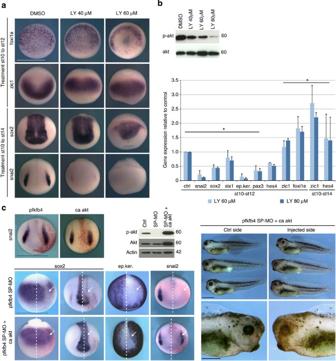Figure 4: Akt signalling mediates PFKFB4 function in ectoderm early patterningin vivo. (a,b) WISH and RT–qPCR analysis showed that pharmacological blockade of PI3K/Akt signallingin vivo, using increasing doses of LY294002, blocked ectoderm specification, while it maintained or increased progenitor marker expression. Three independent experiments were performed and error bars represent s.e.m. (t-test,P≤0.05). Scale bar, 1 mm. (b) Decreased Akt phosphorylation confirmed LY294002 treatment efficiency. (c) PFKFB4 or constitutively active (ca) akt gain-of-functionin vivoproduced very modest expansions of ectoderm territories (heresnail2). PFKFB4 morphant defects were efficiently rescued by ca akt coinjection, allowing normal embryo development, including neurulation and organogenesis. Akt phosphorylation was also restored. Swimming tadpoles developed normally and exhibit beta-galactosidase-labelled progeny of the injected blastomere. Scale bars, 1 mm. Six independent experiments were performed. For WISH, a total of 312 embryos were analysed; the main phenotype is shown and a detailed statistical analysis is given inSupplementary Table 2. Figure 4: Akt signalling mediates PFKFB4 function in ectoderm early patterning in vivo . ( a , b ) WISH and RT–qPCR analysis showed that pharmacological blockade of PI3K/Akt signalling in vivo , using increasing doses of LY294002, blocked ectoderm specification, while it maintained or increased progenitor marker expression. Three independent experiments were performed and error bars represent s.e.m. ( t -test, P ≤0.05). Scale bar, 1 mm. ( b ) Decreased Akt phosphorylation confirmed LY294002 treatment efficiency. ( c ) PFKFB4 or constitutively active (ca) akt gain-of-function in vivo produced very modest expansions of ectoderm territories (here snail2 ). PFKFB4 morphant defects were efficiently rescued by ca akt coinjection, allowing normal embryo development, including neurulation and organogenesis. Akt phosphorylation was also restored. Swimming tadpoles developed normally and exhibit beta-galactosidase-labelled progeny of the injected blastomere. Scale bars, 1 mm. Six independent experiments were performed. For WISH, a total of 312 embryos were analysed; the main phenotype is shown and a detailed statistical analysis is given in Supplementary Table 2 . Full size image Importantly, we then tested the epistasis relationships between PFKFB4 and Akt, as those two enzyme activities have not been associated previously. Constitutively active (ca) akt restored Akt phosphorylation levels in PFKFB4 morphants ( Fig. 4c ). Unilateral coinjection of pfkfb4 morpholino with ca akt mRNA resulted in a spectacular rescue of neural and non-neural markers expression ( Fig. 4c ; Supplementary Fig. 8 ), allowing neural tube closure and further development until tadpole stage ( Fig. 4c ). Both neurulas and swimming tadpoles exhibited healthy lineage-traced cells deriving from the blastomere coinjected with pfkfb4 SP-MO and ca akt. This last result indicated that the mechanism of PFKFB4 critical activity on ectoderm patterning and survival, is mainly dependent on modulating Akt signalling. Apoptosis can be uncoupled from early patterning defects Finally, we confirmed that this novel PFKFB4/Akt function primarily controls ectoderm early patterning and that, if blocked, it secondarily results in cell death. We prevented apoptosis initiation using the antiapoptotic factor Bcl-XL, which acts early in the apoptotic cascade [31] . Bcl-xl mRNA expression in PFKFB4 morphants prevented mid-neurula stage cell death very efficiently, but did not restore neural, neural crest and ectoderm patterning defects ( Supplementary Fig. 6 ). Although we cannot completely rule out the existence of a preapoptotic state in the PFKFB4 morphant cells, this result strongly suggests that the observed early patterning deficiencies are not the consequence of an apoptotic programme initiation, but rather the cause of cell death. Altogether, our results show that PFKFB4/Akt is critical for ectoderm patterning as gastrulation is initiated and that this function cannot be bypassed by adoption of an alternative fate, eventually resulting in cell apoptosis. Our study uncovered a novel function for PFKFB4 in cell fate programming, independent from its classical role in glycolysis regulation. Frog embryo oxidative metabolism allowed experimental uncoupling of glycolysis from other PFKFB4 activities. We showed that PFKFB4 was essential for a novel checkpoint in progenitor cell developmental progression, via Akt signalling (Model, Fig. 5a ). We propose that altering this checkpoint interferes with the cascade of developmental events, causing a developmental arrest: cells remain in a progenitor state. During embryogenesis, when patterning cues are altered, embryonic progenitor cells are diverted towards alternative cell fates, without such arrest: this results in the development of modified but healthy tissues ( Fig. 5b ). Here, the PFKFB4/Akt-linked checkpoint does not alter cell fate equilibrium, but rather acts on all dorsal ectoderm fates simultaneously and allows the developmental progression of progenitor cells: our findings show that Akt is essential for maintaining normal development ( Fig. 5c ). We propose that the arrest in development of progenitors, that cannot be resolved, then activates apoptotic elimination of the defective cells. The molecular link between PFKFB4 and Akt signalling remains elusive. Coimmunoprecipitation experiments failed to pull down a protein complex ( Supplementary Fig. 7 ), suggesting indirect relationships. Further studies will explore the nature of these interactions that may involve non-conventional activities for PFKFB4 or interactions between PFKFB4 and upstream regulators of Akt. 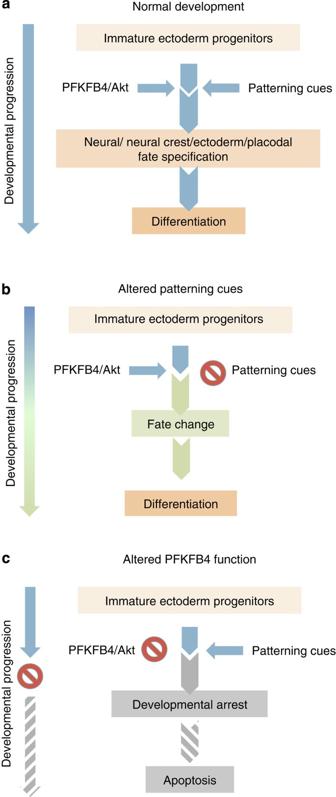Figure 5: Model of PFKFB4 function during embryonic patterning. We propose that, during normal development, (a) PFKFB4/Akt-linked checkpoint allows developmental progression and patterning to occur. (b) If patterning signals are altered, it is known that developing progenitors follow alternative fates. (c) In contrast, if PFKFB4/Akt pathway is defective, no viable developmental alternative is offered to progenitor cells, which arrest their developmental programme at progenitor stage and eventually undergo apoptosis. Figure 5: Model of PFKFB4 function during embryonic patterning. We propose that, during normal development, ( a ) PFKFB4/Akt-linked checkpoint allows developmental progression and patterning to occur. ( b ) If patterning signals are altered, it is known that developing progenitors follow alternative fates. ( c ) In contrast, if PFKFB4/Akt pathway is defective, no viable developmental alternative is offered to progenitor cells, which arrest their developmental programme at progenitor stage and eventually undergo apoptosis. Full size image Whereas numerous studies highlight the importance of metabolic regulations in various normal and pathological cell processes [1] , [2] , [3] , [4] , [5] , [6] , [32] , [33] , [34] , [35] , [36] , few studies have explored novel roles of classical metabolism regulators [4] , [37] . Our results demonstrate that normal, cytoplasmic, PFKFB4 levels are a prerequisite for ectoderm development and survival. The enrichment of pfkfb4 expression in frog and chick dorsal ectoderm during gastrulation and neurulation suggested that these cells might display an acute sensitivity to PFKFB4/Akt levels during their early specification, although other cell types that express lower levels of pfkfb4 or other pfkfb isoforms, may also respond to similar regulations. In addition, it will be interesting to compare this novel PFKFB4/Akt signalling to PI3K/Akt/GSK3 signalling affecting early dorsal axis formation during cleavage stages [38] . Future work will address PFKFB/Akt signalling mechanisms, in dorsal ectoderm and other contexts of stem cell differentiation. All reagents are listed in Supplementary Table 1 . Sample size is chosen to be statistically significant, at least three independent experiments are conducted for each condition, series of injected embryos are at least of 20 embryos. All phenotypes shown are the most frequent phenotype for each experiment. All details on the statistical analysis and total sample counts are given in Supplementary Table 2 . Embryo injections Xenopus laevis and Gallus gallus embryos were obtained, staged and dissected using standard procedures [39] , [40] . The care and use of animals used here was strictly applying European and National Regulation for the Protection of Vertebrate Animals used for Experimental and other Scientific Purposes in force (facility licence #C91-471-108 given by the Direction Départementale de Protection de la Population, Courcouronnes, France). X. laevis embryos were obtained by in vitro fertilization using standard procedures and were staged according to Niewkoop and Faber developmental table [39] , [41] . For in vivo analysis, embryos were injected unilaterally at four-cell stage and grown until stages 10–40. Nuclear-targeted beta-galactosidase mRNA was coinjected as a lineage tracer with each mRNA or MOs. Beta-galactosidase activity was revealed in red, indicating the injected side, before WISH. For whole-embryo injections, the two blastomeres were injected at two-cell stage in the animal pole. Animal cap explants were cut at blastula stage 9 and dorsal explants at either late gastrula stage 12 or mid-neurula stage 14. mRNAs used for microinjection were obtained by in vitro transcription of plasmids containing the desired cDNA using the mMessage mMachine SP6 or T7 kits (Ambion) and purified on G50 sephadex spin columns. The following plasmids were used: bcl-xl [42] , ca akt [43] , memcherry [44] , nlacZ [45] , noggin [46] , pfkfb4 (this study), pfkfb4–gfp (this study) and tcf3VP16-GR [47] . PFKFB4 silencing was performed using translation-blocking or splice-blocking antisense morpholino oligonucleotides (GeneTools, this study). The efficiency and specificity of the MOs was tested by 35 S-labelled in vitro transcription-and-translation reaction using TNT kit (Promega) or RT–qPCR. Reagents, plasmids and morpholinos are further described in Supplementary Table 1 . Whole-mount in situ hybridization (WISH) Embryos were fixed and prepared for WISH according to a fast protocol optimized for superficial structures [48] . Antisense digoxygenin-labelled RNA probes were used at a final concentration of 1 μg ml −1 . The following probes were used: ep. ker . [49] , foxi1e [50] , hes4 (ref. 51 ), myod [52] , pax3 (ref. 26 ), X. laevis pfkfb4 (this study), chick pfkfb4 (this study), six1 (ref. 53 ), snai2 (ref. 54 ), sox10 (ref. 55 ) and zic1 (ref. 56 ). All NCBI Reference Sequences are listed in Supplementary Table 1 . Additional pictures showing groups of embryos are presented in Supplementary Fig. 8 . Coimmunoprecipitation and western blotting Immunoprecipitation and western blot analysis were performed as previously described [57] . In brief, lysates of HEK293T or 5–10 embryos were prepared with cold lysis buffer. Immunoprecipitations were conducted on HEK293T cell lysates at 4 °C for 3 h with anti-HA antibody and protein-A sepharose beads (Sigma). Immunoprecipitates were washed with lysis buffer three times and analysed by western blot. All antibodies were diluted in 5% skimmed milk. The concentration and source of all antibodies used for western blotting are detailed in Supplementary Table 1 . Full scans of blots accompanied by the position of molecular weight markers are shown in Supplementary Fig. 9 . Semi-quantitative and RT–qPCR Embryos were lysed in proteinase K-containing lysis buffer, followed by DNAse treatment and reverse transcription [39] . RT–qPCR was performed according to standard procedures using MIQE recommendations. Ef1α and odc were used as controls. Results are shown relative to expression in sibling control samples. The sequences of all primers used in this study are listed in Supplementary Table 1 . Glycolysis measurement GAPDH activity and lactate concentration were measured on lysates from 20 sibling embryos using KD-Alert GAPDH kit (Life Technologies) and L-Lactate Kit (Abcam). Cell death Embryos were fixed in 3.7% formaldehyde in PBS and dehydrated in methanol. Apoptotic cells were visualized using acridine orange staining or cleaved caspase-3 immunostaining [42] . The concentration and source of reagents and antibodies are detailed in Supplementary Table 1 . Imaging Confocal images were obtained from cryosections of embryos expressing PFKFB4–GFP, GFP or memCherryFP (Leica SP5, 60X/1.4) [58] . Subcellular GFP fluorescence (in pixel intensities) was measured on a total of 60 cells per condition (ImageJ software). How to cite this article : Pegoraro, C. et al . PFKFB4 controls embryonic patterning via Akt signalling independently of glycolysis. Nat. Commun. 6:5953 doi: 10.1038/ncomms6953 (2015).